Nutritional stress induces exchange of cell material and energetic coupling between bacterial species Knowledge of the behaviour of bacterial communities is crucial for understanding biogeochemical cycles and developing environmental biotechnology. Here we demonstrate the formation of an artificial consortium between two anaerobic bacteria, Clostridium acetobutylicum (Gram-positive) and Desulfovibrio vulgaris Hildenborough (Gram-negative, sulfate-reducing) in which physical interactions between the two partners induce emergent properties. Molecular and cellular approaches show that tight cell–cell interactions are associated with an exchange of molecules, including proteins, which allows the growth of one partner ( D. vulgaris ) in spite of the shortage of nutrients. This physical interaction induces changes in expression of two genes encoding enzymes at the pyruvate crossroads, with concomitant changes in the distribution of metabolic fluxes, and allows a substantial increase in hydrogen production without requiring genetic engineering. The stress induced by the shortage of nutrients of D. vulgaris appears to trigger the interaction. Bacteria have usually been studied in single culture in rich media or in specific starvation conditions. These studies have contributed to understanding and characterizing their metabolism. However, they coexist in nature with other microorganisms and form consortia in which they interact to build an advanced society [1] that drives key biogeochemical cycles [2] . These consortia vary in space and time as a function of the nutrients [3] , [4] . In such microbial networks, microorganisms can develop different types of interaction, such as exchange of metabolites. The observed phenotype results from these interactions and not from the individual genotypes alone [5] . The interaction with other species allows microorganisms to occupy environmental niches that would otherwise be closed to them and, depending on the ecological niche occupied, they can show different properties and functions. Mixed cultures have accordingly broader metabolic capabilities and greater robustness to environmental fluctuations than single cultures, characteristics that are attractive for biotechnology [6] , [7] . However, our knowledge of the physical and metabolic interactions that help microbes to survive and to develop in a complex network is limited. In anaerobic environments microorganisms cooperate in the feeding chains, and the complete degradation of complex matter to methane and carbon dioxide (CO 2 ) involves at least four groups of microorganisms, including primary and secondary fermenters and at least two types of methanogenic archaea [8] . Many studies have examined the syntrophic growth of sulfate-reducing bacteria (SRB) acting like secondary fermenters and methanogenic archaea [9] , [10] , [11] . Most recently, the metabolic interaction between Clostridia, acting as primary fermenters, and methanogenic archaea has also been studied [12] , [13] , highlighting a symbiotic process of interspecies hydrogen transfer that does not require physical interaction. However, very few studies have examined interaction between SRB and Clostridia, and little is known about the complex interactions that occur in natural bacterial consortia and how primary fermenter bacteria such as Clostridia compete with other anaerobes like SRB [8] . We have accordingly constructed an artificial consortium constituted by Desulfovibrio vulgaris Hildenborough and Clostridium acetobutylicum . These bacteria are representative of species found in the same environment and are both involved in biomass degradation [8] . D. vulgaris Hildenborough is a Gram-negative SRB that uses sulfate as a terminal electron acceptor for the heterotrophic oxidation of organic compounds or hydrogen (H 2 ) to produce sulfide [14] . C. acetobutylicum is a strictly fermentative endospore-forming Gram-positive bacterium. It converts sugars and starch to organic acids (acetate, butyrate and lactate) during acidogenesis and solvents (acetone and butanol) during solventogenesis [15] , [16] , [17] . Here we show that the condition of nutriment starvation for D. vulgaris in the co-culture induces interspecies cell–cell interaction, allowing exchange of cytoplasmic material (tested with fluorescent molecules, including proteins), associated with metabolic changes and much higher production of H 2 . The metabolic changes suggest that the understanding of microbial consortia may offer a type of ecological engineering of microbial ecosystems that could provide new approaches for modifying or controlling metabolic pathways. Physical contact is needed for growth of D. vulgaris We defined a medium (GY) that allowed growth of C. acetobutylicum and survival of D. vulgaris . Both the strains have been grown on their classical media (Starkey medium for D. vulgaris and 2YTG medium for C. acetobutylicum ), and then washed three times before inoculation. Strikingly, when the two strains were present together, maximum growth (estimated by optical density) occurred earlier than seen for growth of C. acetobutylicum in a pure culture ( Fig. 1a ). The growth pattern follows glucose consumption ( Fig. 1b ). As expected, there was no growth of D. vulgaris in single culture, in GY medium, as D. vulgaris cannot grow on glucose or other hexoses, because of lack of permeases [18] . Survival of D. vulgaris in single culture in GY medium can be explained by its capacity to accumulate and to use polyglucose and elemental sulfur particles when necessary [19] . Its capacity to use sulfur particles was confirmed by the production of H 2 S at a concentration of 0.15 mM (at the end of the exponential phase), higher than that of 0.035 mM sulfate derived from the inorganic nutrients and yeast extract present in the GY medium. The coexistence of the two bacteria in the co-culture in GY medium was assessed using specific gene markers and cell viability experiments ( Supplementary Fig. 1 ). The growth of C. acetobutylicum and D. vulgaris in the co-culture was confirmed by flow cytometry, taking advantage of their difference in shape ( Supplementary Fig. 2 ). In addition, dynamics of the two strains in the co-culture were monitored with quantitative PCR (qPCR). 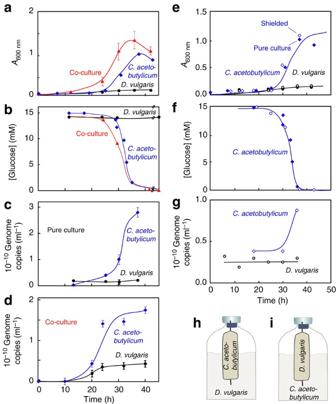Figure 1: Growth ofD. vulgarisandC. acetobutylicumin co-culture on GY medium. (a) Absorbance curves forD. vulgarisin pure culture,C. acetobutylicumin pure culture and co-culture, as indicated. (b) Glucose consumption in the two pure cultures and the co-culture. (c,d) Numbers of genome copies in pure culture (c) and co-culture (d) as a function of time. The numbers of genome copies of each strain were determined by qPCR, using thedsrAgene forD. vulgarisand theendoGgene forC. acetobutylicum.Notice that the pure culture ofD. vulgarisdoes not consume glucose and does not grow. The right-hand panels show experiments in which open symbols represent bacteria shielded from one another by a dialysis membrane, and filled symbols represent results in pure cultures with no shielding. (e) Absorbance curves forD. vulgarisshielded fromC. acetobutylicumand forC. acetobutylicumshielded fromD. vulgaris. Controls of pure cultures are also shown. (f) Glucose consumption ofC. acetobutylicumshielded fromD. vulgaris, with a control ofC. acetobutylicumin pure culture. (g) Numbers of genome copies determined as inc. (h,i) Illustration of the experimental set-ups: (h) for the curves related to shieldedD. vulgarisand (i) for the ones related to shieldedC. acetobutylicum.Results are means±s.d. (n=3). Figure 1c,d highlights the fact that D. vulgaris grows only in the presence of C. acetobutylicum , as the number of genome copies increases with time. As expected, C. acetobutylicum grows both in single culture and in co-culture. The progressive formation of cell aggregates may explain why in Supplementary Fig. 2a there is only one peak at 30 h. Figure 1: Growth of D. vulgaris and C. acetobutylicum in co-culture on GY medium. ( a ) Absorbance curves for D. vulgaris in pure culture, C. acetobutylicum in pure culture and co-culture, as indicated. ( b ) Glucose consumption in the two pure cultures and the co-culture. ( c , d ) Numbers of genome copies in pure culture ( c ) and co-culture ( d ) as a function of time. The numbers of genome copies of each strain were determined by qPCR, using the dsrA gene for D. vulgaris and the endoG gene for C. acetobutylicum. Notice that the pure culture of D. vulgaris does not consume glucose and does not grow. The right-hand panels show experiments in which open symbols represent bacteria shielded from one another by a dialysis membrane, and filled symbols represent results in pure cultures with no shielding. ( e ) Absorbance curves for D. vulgaris shielded from C. acetobutylicum and for C. acetobutylicum shielded from D. vulgaris . Controls of pure cultures are also shown. ( f ) Glucose consumption of C. acetobutylicum shielded from D. vulgaris , with a control of C. acetobutylicum in pure culture. ( g ) Numbers of genome copies determined as in c . ( h , i ) Illustration of the experimental set-ups: ( h ) for the curves related to shielded D. vulgaris and ( i ) for the ones related to shielded C. acetobutylicum. Results are means±s.d. ( n =3). Full size image To better understand the growth of D. vulgaris in the co-culture, we tested whether D. vulgaris could use the metabolites produced by C. acetobutylicum , and whether their presence would allow D. vulgaris growth. C. acetobutylicum was grown in the GY medium, and at various times cells were removed and a washed suspension of D. vulgaris was inoculated. No D. vulgaris growth was detected after 30 h, at any ratio of glucose to metabolite products, suggesting that D. vulgaris cannot use the metabolites produced, even when it was inoculated after 36 h of C. acetobutylicum growth, when the butyrate concentration was 7.7 mM, the acetate concentration 4.6 mM and the lactate concentration 2.3 mM (and no glucose). Furthermore, the addition of 20 mM lactate to the GY medium does not allow the growth of D. vulgaris in pure culture ( Supplementary Table 1 ). The presence of C. acetobutylicum cells appears necessary for the growth of D. vulgaris. It could be argued, however, that in these experiments the H 2 and the CO 2 produced by C. acetobutylicum had been lost. The two bacteria were accordingly co-cultivated with either D. vulgaris or C. acetobutylicum confined in a dialysis tube ( Fig. 1h,i ), which prevents physical interspecies interaction but not the diffusion of small molecules, such as the metabolites or small proteins (<7 kDa). Whether D. vulgaris was in the dialysis tube or outside, there was no growth ( Fig. 1e,g ); the culture behaved like pure D. vulgaris culture. When C. acetobutylicum was in the outside medium and D. vulgaris in the dialysis bag ( Fig. 1i ), the growth profile of C. acetobutylicum was not significantly altered in relation to the pure culture ( Fig. 1e,g ); there was no modification in glucose consumption either ( Fig. 1f ). These experiments suggest that the growth of D. vulgaris requires the two bacteria to be present in the same compartment and most probably in conditions that allow cell–cell interaction, as the element that allows D. vulgaris growth appears not to be freely diffusible through a dialysis membrane. In the absence of yeast extract in the culture medium, there was no growth with any of the pure cultures. The co-culture however presented a small but significant growth ( Supplementary Table 1 ). This suggests, as proposed by Kato [20] in the case of syntrophic co-culture of Pelotomaculum thermopropionicum and Methanothermobacter thermautotrophicus , that amino acids and coenzymes can be transferred between C. acetobutylicum and D. vulgaris . Exchange of cytoplasmic molecules between the bacteria Networks of bacterial cells were observed in the co-culture ( Supplementary Fig. 3 ) and the occurrence of physical contact between the two strains was confirmed by flow cytometry ( Supplementary Fig. 2 ). A possible non-specific aggregation of the two bacteria, a well known phenomenon [21] , can be ruled out as no co-aggregation is observed in the pure cultures as the peaks are not displaced ( Supplementary Fig. 2 ) or when the two pure cultures are mixed, unlike for Myxococcus xanthus [22] when aggregate appeared. The physical interaction between D. vulgaris and C. acetobutylicum in the co-culture was further investigated by fluorescence microscopy. As D. vulgaris is Gram-negative and C. acetobutylicum Gram-positive with an external wall of peptidoglycan, the co-culture was labelled with fluorochromes to specifically mark the cytoplasmic membrane (red fluorescence) and peptidoglycan wall (green fluorescence) ( Supplementary Fig. 4 ). Fluorescence microscopy revealed zones where the two bacteria interacted, these being apparently associated with a decrease in the green fluorescence (marker of peptidoglycan), suggesting either a partial loss of peptidoglycan after the interaction or an interaction where peptidoglycan was missing ( Supplementary Fig. 4b ). However, the possibility that the decrease in fluorescence is due to differences in the focal planes of the cells cannot be ruled out. This interaction was further analysed by the scanning electron microscopy (SEM) ( Fig. 2 ). Conglomerates of the two types of bacteria were again observed in the co-culture ( Fig. 2c ) and in some cases, cell–cell interactions ( Fig. 2d ) are reminiscent of those described by Dubey [23] . 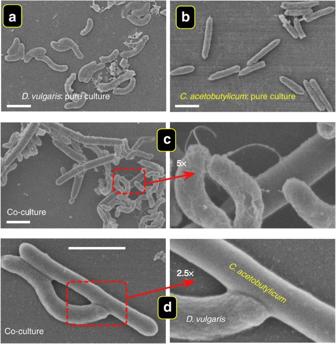Figure 2: Scanning electron microscopy ofD. vulgarisandC. acetobutylicumin pure culture and co-culture. Exponentially growingC. acetobutylicumin 2YTG medium orD. vulgarisin Starkey medium under anaerobic conditions was diluted in fresh GY medium (forC. acetobutylicum) or fresh Starkey medium (forD. vulgaris), and transferred to Hungate tubes containing coverslips. For the co-culture, GY medium was used, and the bacteria were washed in GY medium before the co-culture. In all three cases, the coverslips were removed after 30-h growth, fixed with glutaraldehyde, dried chemically with hexamethyldisilane and coated with gold–palladium particles with a FINE COAT-ion sputter JFC 1100. Digital images were acquired with the NEWTEC system. (a,b) Images ofD. vulgarisin the Starkey medium (a) andC. acetobutylicumin GY medium (b) in pure cultures. (c) Images of the two bacteria in co-culture. (d) Image of aD. vulgariscell in close contact with aC. acetobutylicumcell. Images of the boxed regions are shown at higher magnification at the right. Scale bar, 1 μm in all panels. Figure 2: Scanning electron microscopy of D. vulgaris and C. acetobutylicum in pure culture and co-culture. Exponentially growing C. acetobutylicum in 2YTG medium or D. vulgaris in Starkey medium under anaerobic conditions was diluted in fresh GY medium (for C. acetobutylicum ) or fresh Starkey medium (for D. vulgaris ), and transferred to Hungate tubes containing coverslips. For the co-culture, GY medium was used, and the bacteria were washed in GY medium before the co-culture. In all three cases, the coverslips were removed after 30-h growth, fixed with glutaraldehyde, dried chemically with hexamethyldisilane and coated with gold–palladium particles with a FINE COAT-ion sputter JFC 1100. Digital images were acquired with the NEWTEC system. ( a , b ) Images of D. vulgaris in the Starkey medium ( a ) and C. acetobutylicum in GY medium ( b ) in pure cultures. ( c ) Images of the two bacteria in co-culture. ( d ) Image of a D. vulgaris cell in close contact with a C. acetobutylicum cell. Images of the boxed regions are shown at higher magnification at the right. Scale bar, 1 μm in all panels. Full size image The tight cell–cell interactions suggested the possibility of intercellular exchange of molecules. This was investigated using calcein-labelled D. vulgaris or C. acetobutylicum , as described in Material and Methods. When D. vulgaris was incubated in Starkey medium with calcein–acetoxymethyl (AM) ester, a strong green fluorescence was observed after 2-h incubation at 37 °C indicating calcein sequestration in the cytoplasm. Fluorescent D. vulgaris was washed, mixed with unlabelled C. acetobutylicum and the mixture was directly visualized by fluorescence microscopy or diluted in fresh GY medium. At time zero, only D. vulgaris was fluorescent ( Fig. 3a ), but after 24 h, a fluorescence signal was observed from C. acetobutylicum in interaction with D. vulgaris ( Fig. 3b and Supplementary Fig. 5a , which illustrates a bigger field). However, C. acetobutylicum cells not in contact with D. vulgaris display little or no fluorescence ( Fig. 3c ). The response was displayed by 80–90% of C. acetobutylicum cells (percentages estimated from multiple random fields in three separate biological replicates). There was a similar transfer of fluorescence with calcein-labelled C. acetobutylicum mixed with unlabelled D. vulgaris ( Fig. 3d,e and Supplementary Fig. 5b ). Thus, calcein can be transferred between C. acetobutylicum cytoplasm and D. vulgaris in either direction. 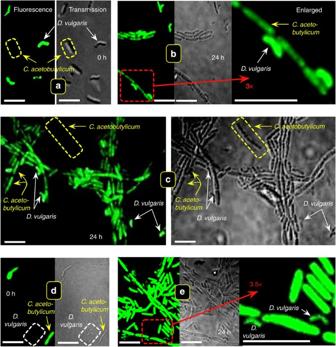Figure 3: Exchange of calcein betweenD. vulgarisandC. acetobutylicum. D. vulgarisgrowing exponentially in Starkey medium was labelled with calcein, washed with GY medium, mixed with unlabelledC. acetobutylicumand visualized by fluorescence confocal microscopy at time zero (a) or after 24-h incubation at 37 °C in GY medium (b). (c) A bigger field. (d,e) Exponentially growingC. acetobutylicumlabelled with calcein was washed, mixed with unlabelledD. vulgarisand visualized at time zero (d) or after 24-h incubation at 37 °C in GY medium (e). Non-fluorescent cells are in yellow or white boxes, as labelled. Scale bar, 2 μm. Figure 3: Exchange of calcein between D. vulgaris and C. acetobutylicum . D. vulgaris growing exponentially in Starkey medium was labelled with calcein, washed with GY medium, mixed with unlabelled C. acetobutylicum and visualized by fluorescence confocal microscopy at time zero ( a ) or after 24-h incubation at 37 °C in GY medium ( b ). ( c ) A bigger field. ( d , e ) Exponentially growing C. acetobutylicum labelled with calcein was washed, mixed with unlabelled D. vulgaris and visualized at time zero ( d ) or after 24-h incubation at 37 °C in GY medium ( e ). Non-fluorescent cells are in yellow or white boxes, as labelled. Scale bar, 2 μm. Full size image To test whether the two bacteria could exchange larger molecules than calcein, such as proteins, we examined whether D. vulgaris could exchange mCherry molecules (or green fluorescent protein, GFP) with C. acetobutylicum . For that purpose, D. vulgaris harbouring a pRD3 plasmid containing the gene mCherry that codes for mCherry was mixed with C. acetobutylicum cells lacking the mCherry gene but labelled with calcein, and the co-culture was analysed by microscopy. At time zero, C. acetobutylicum shows a green fluorescence and D. vulgaris a red fluorescence ( Fig. 4a ), but after 24 h, both the bacteria show both green and red fluorescence, indicating the presence of mCherry in C. acetobutylicum and calcein in D. vulgaris ( Fig. 4a ). 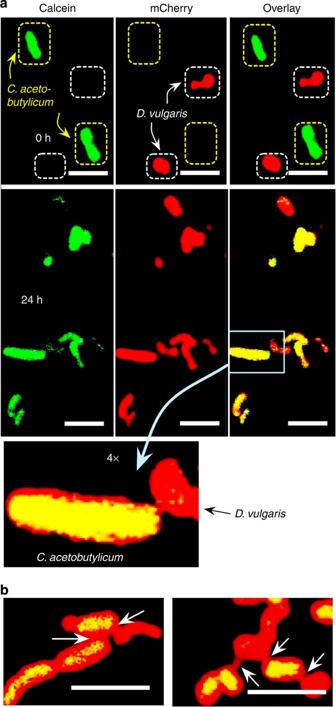Figure 4: Bidirectional transfer of calcein and mCherry betweenC. acetobutylicumandD. vulgaris. (a)D. vulgarisgrowing exponentially in Starkey medium was labelled with mCherry (red), washed in GY medium, mixed withC. acetobutylicumlabelled with calcein (green) and visualized by fluorescence confocal microscopy at time zero or after 24-h incubation at 37 °C in GY medium. Notice that at time zero, each type of bacteria shows only green or red fluorescence, but after 24 h,C. acetobutylicumoriginally green, shows red fluorescence, andD. vulgarisoriginally red, shows green fluorescence. (b) Results from an equivalent experiment showing exchange of fluorescent labels in both directions (yellow). White arrows indicate apparent connections between bacterial cells. Scale bar, 2 μm in all panels. Figure 4b illustrates results from another equivalent experiment, and the white arrows point to the connections between C. acetobutylicum and D. vulgaris ; these connecting structures in Fig. 4a,b are consistent with the SEM images. Figure 4: Bidirectional transfer of calcein and mCherry between C. acetobutylicum and D. vulgaris . ( a ) D. vulgaris growing exponentially in Starkey medium was labelled with mCherry (red), washed in GY medium, mixed with C. acetobutylicum labelled with calcein (green) and visualized by fluorescence confocal microscopy at time zero or after 24-h incubation at 37 °C in GY medium. Notice that at time zero, each type of bacteria shows only green or red fluorescence, but after 24 h, C. acetobutylicum originally green, shows red fluorescence, and D. vulgaris originally red, shows green fluorescence. ( b ) Results from an equivalent experiment showing exchange of fluorescent labels in both directions (yellow). White arrows indicate apparent connections between bacterial cells. Scale bar, 2 μm in all panels. Full size image A similar experiment, but using unlabelled C. acetobutylicum , was done with D. vulgaris harbouring a pRD2 plasmid containing the gene gfp that codes for GFP. At time zero, only D. vulgaris shows green fluorescence, but after 24 h, a green fluorescence from C. acetobutylicum was also observed, indicating the presence of GFP in C. acetobutylicum and in D. vulgaris ( Supplementary Fig. 6 ). The possibility that the red fluorescence associated with C. acetobutylicum would be due to acquisition of the pRD3 plasmid from D. vulgaris through conjugation can be ruled out, as C. acetobutylicum strain ATCC824 contains a Cac824I restriction endonuclease, which prevents transformation of C. acetobutylicum with shuttle vectors used in other bacteria [24] , [25] . The pRD3 and pRD2 plasmids used in our study contain many Cac824I sites [26] and in consequence they are unstable in C. acetobutylicum . This supports the view that the fluorescence associated with C. acetobutylicum cells is due to the transfer of mCherry or GFP from D. vulgaris to C. acetobutylicum . When the experiments with calcein–AM ester were repeated with either D. vulgaris or C. acetobutylicum confined in the dialysis tube to prevent physical interspecies interaction (as in Fig. 1h,i ), there was no fluorescence transfer after 24 h ( Fig. 5a,b ), indicating that the fluorescent molecules cannot enter or leave the cells via the medium culture. 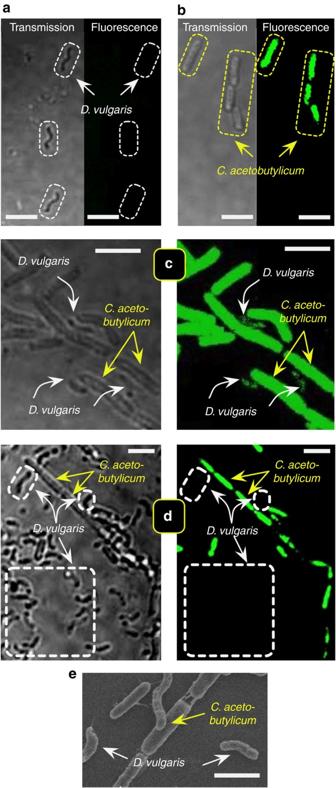Figure 5: Effect of various conditions on transfer of calcein from labelledC. acetobutylicumto D. vulgaris. All results are shown after 24 h of co-culture, and in all panels the scale bars, 2 μm. (a) No transfer whenC. acetobutylicumis shielded fromD. vulgarisby a dialysis membrane and cultivated in GY medium at 37 °C (D. vulgarisshows no fluorescence) and (b) theC. acetobutylicumremains labelled. (c) Transfer of calcein fromC. acetobutylicumtoD. vulgarisin co-culture in GY medium supplemented with 20 mM lactate (without shielding). (d) No transfer observed in GY medium supplemented with 20 mM sulfate in addition to 20 mM lactate. A great number ofD. vulgariscells (which can grow on sulfate) can be seen, but they show no green fluorescence, indicating that the transfer has been greatly reduced (or is non-existent). (e) A scanning electron micrograph made in the same conditions as (d). Scale bar, 2 μm in all panels. Figure 5: Effect of various conditions on transfer of calcein from labelled C. acetobutylicum to D . vulgaris. All results are shown after 24 h of co-culture, and in all panels the scale bars, 2 μm. ( a ) No transfer when C. acetobutylicum is shielded from D. vulgaris by a dialysis membrane and cultivated in GY medium at 37 °C ( D. vulgaris shows no fluorescence) and ( b ) the C. acetobutylicum remains labelled. ( c ) Transfer of calcein from C. acetobutylicum to D. vulgaris in co-culture in GY medium supplemented with 20 mM lactate (without shielding). ( d ) No transfer observed in GY medium supplemented with 20 mM sulfate in addition to 20 mM lactate. A great number of D. vulgaris cells (which can grow on sulfate) can be seen, but they show no green fluorescence, indicating that the transfer has been greatly reduced (or is non-existent). ( e ) A scanning electron micrograph made in the same conditions as ( d ). Scale bar, 2 μm in all panels. Full size image No nutrient known to be used by D. vulgaris was present in the GY culture medium in any of the exchange experiments ( Figs 3 and 4 ). Addition of lactate (20 mM) alone, a fermentative substrate for D. vulgaris , did not modify significantly the behaviour of the co-culture ( Supplementary Table 1 ), and calcein fluorescence transfer from C. acetobutylicum to D. vulgaris was still observed after 24 h of co-culture ( Fig. 5c ). However addition to the culture medium of lactate (20 mM), used as electron donor and carbon source and sulfate (20 mM, electron acceptor) which allows sulfur respiration metabolism in D. vulgaris , prevents or at least greatly reduced the interspecies molecular exchange, as there appears to be no transfer of fluorescence in this case ( Fig. 5d ). No tight contact similar to that observed without lactate and sulfate ( Fig. 2 ) was detected by SEM ( Fig. 5e ). These results support the hypothesis that the cell–cell interactions and material transfer are a response to the starvation conditions of D. vulgaris. The fact that lactate alone does not inhibit the transfer means that D. vulgaris cannot use this nutriment properly, as could be expected in view of the high H 2 concentration present, and in consequence the starvation conditions persist. Control experiments show that lactate, sulfate or both have no effect on single culture of C. acetobutylicum ( Supplementary Table 1 ). The hypothesis that the shortage of nutrients can be the triggering factor for the cytoplasmic exchange was explored further by the experiments with Escherichia coli labelled with mCherry and co-cultivated with either C. acetobutylicum ( Fig. 6 ) or D. vulgaris ( Fig. 7 ) labelled with calcein. In co-culture of E. coli plus C. acetobutylicum , both the bacteria grew, but in contrast to what was observed with D. vulgaris and C. acetobutylicum , no interaction and no exchange of fluorescent molecules was observed ( Fig. 6 ). In this case there is no nutritional stress for either of the bacteria as E. coli can use glucose for its growth. This suggests that bacterial interactions in synthetic microbial consortia may emerge as a consequence of individual species solving their own problems of allocation of metabolic resources. Furthermore, this conclusion is supported by the co-culture experiment of E. coli plus D. vulgaris , ( Fig. 7 ), where the two bacteria grew and interact together, with exchange of fluorescent molecules. Notice the great quantity of bacteria that contain both labels (yellow) illustrated in Fig. 7b . 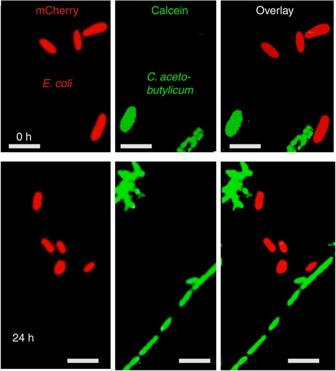Figure 6: Absence of exchange of fluorescent molecules betweenE. coliandC. acetobutylicum. (a) Exponentially growingC. acetobutylicumlabelled with calcein (green) was mixed withE. colilabelled with mCherry (red), and the mixture was visualized by fluorescence confocal microscopy at time zero or after 24 h of incubation at 37 °C. Notice that in contrast toFig. 4, no yellow colour can be seen in the overlay and noC. acetobutylicumshows red fluorescence. Scale bar, 2 μm in all panels. Figure 6: Absence of exchange of fluorescent molecules between E. coli and C. acetobutylicum . ( a ) Exponentially growing C. acetobutylicum labelled with calcein (green) was mixed with E. coli labelled with mCherry (red), and the mixture was visualized by fluorescence confocal microscopy at time zero or after 24 h of incubation at 37 °C. Notice that in contrast to Fig. 4 , no yellow colour can be seen in the overlay and no C. acetobutylicum shows red fluorescence. Scale bar, 2 μm in all panels. 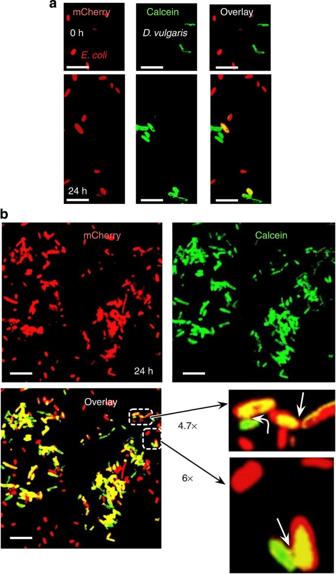Figure 7: Exchange of fluorescent molecules betweenE. coliandD. vulgaris. (a) Exponentially growingD. vulgarislabelled with calcein (green) was washed with GY medium, mixed withE. colilabelled with mCherry (red), and the mixture was visualized at time zero or after 24-h incubation at 37 °C. Yellow colour, indicating exchange of both labels, is visible in the overlay. (b) A similar experiment with a bigger field. Notice the many cells with both labels (yellow). The white arrows indicate connections betweenE. coliandD. vulgaris. Scale bar, 2 μm in all panels. Full size image Figure 7: Exchange of fluorescent molecules between E. coli and D. vulgaris . ( a ) Exponentially growing D. vulgaris labelled with calcein (green) was washed with GY medium, mixed with E. coli labelled with mCherry (red), and the mixture was visualized at time zero or after 24-h incubation at 37 °C. Yellow colour, indicating exchange of both labels, is visible in the overlay. ( b ) A similar experiment with a bigger field. Notice the many cells with both labels (yellow). The white arrows indicate connections between E. coli and D. vulgaris . Scale bar, 2 μm in all panels. Full size image Modification of H 2 metabolism in the co-culture In the co-culture, as well as in the single C. acetobutylicum culture, the growth and production of metabolites resulted from the complete consumption of glucose ( Figs 1b and 8a ). More than 90% of the electron equivalents were recovered ( Supplementary Fig. 7 ). This suggests that all the main metabolites have been detected, and that any others that could have been produced were at concentrations below the detection threshold, and consequently negligible as carbon sources, although they could still act as signals. No solvents (ethanol, acetone and butanol) were detected except occasionally in very small amounts. This observation is in agreement with the experimental conditions used, as production of solvents occurs at much higher concentrations of glucose (typically around 500 mM, much more than the 14 mM used in our experiments), when the pH is lower (4.5 instead of 5.5 in our experiments) and when acids are reassimilated in the stationary phase, which occurs only when acid concentrations are at least around 60 mM [27] . 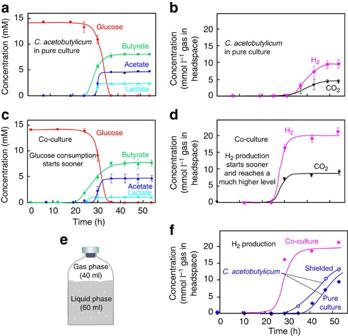Figure 8: Time courses of glucose consumption and metabolite production of pure culture ofC. acetobutylicumand co-culture. (a) Consumption of glucose, and production of butyrate, acetate and lactate in pure culture. (b) Production of H2and CO2. (c) Consumption of glucose and production of anions in co-culture. (d) Production of gases in co-culture. (e) Schematic representation of the Hungate tube used for the culture. (f) Production of H2byC. acetobutylicumin pure culture, in co-culture and shielded (withD. vulgarisin a dialysis tube, as inFig. 1i), as labelled. Results are means±s.d. (n=3). Figure 8: Time courses of glucose consumption and metabolite production of pure culture of C. acetobutylicum and co-culture. ( a ) Consumption of glucose, and production of butyrate, acetate and lactate in pure culture. ( b ) Production of H 2 and CO 2 . ( c ) Consumption of glucose and production of anions in co-culture. ( d ) Production of gases in co-culture. ( e ) Schematic representation of the Hungate tube used for the culture. ( f ) Production of H 2 by C. acetobutylicum in pure culture, in co-culture and shielded (with D. vulgaris in a dialysis tube, as in Fig. 1i ), as labelled. Results are means±s.d. ( n =3). Full size image Single culture of D. vulgaris did not consume glucose ( Fig. 1b ) and no metabolites were detected, in agreement with absence of growth. The same organic acids, that is, lactate, acetate and butyrate, were detected and in similar concentrations in the pure C. acetobutylicum culture and in the co-culture, except for the lactate concentration, which decreased by half in the co-culture: this could imply more reducing power for H 2 production. In line with this possibility, the concentrations of H 2 and CO 2 in the co-culture were substantially higher ( Fig. 8b,d ), with a H 2 yield about three times that of the single culture, reaching 3.46 mol H 2 mol −1 of glucose consumed. Due to the high concentration of H 2 in the co-culture, the alternative possibility of H 2 production by D. vulgaris via lactate (produced by C. acetobutylicum ) fermentation is not probable [28] and in addition there was no growth of D. vulgaris in pure culture in the GY medium supplemented with 20 mM lactate ( Supplementary Table 1 ). The fact that the H 2 /CO 2 ratio was rather similar in single culture or co-culture suggests an unchanged flux distribution between acetate and butyrate pathways in C. acetobutylicum . To get insight into the metabolic changes in C. acetobutylicum in the co-culture, reverse transcription PCR was applied to specific genes coding for lactate dehydrogenase ( ldh ) and pyruvate ferredoxin oxidoreductase ( pfor ), the enzymes in the branch point of pyruvate ( Supplementary Fig. 8 ). Changes in their relative activities can alter the flux distribution and thus vary H 2 production. Gene expression studies showed that at 30 h of growth of the co-culture, expression of the pfor gene considerably increased by a factor of 6.5±0.5, whereas the ldh gene was downregulated by a factor of 0.3±0.1 (comparison between single culture and co-culture). Assuming that the enzyme activities are proportional to the amounts of messenger RNA, this could produce higher flux distribution from pyruvate to acetyl-CoA than to lactate, thereby increasing the amount of reduced ferredoxin necessary for the H 2 production. The substantial upregulation of the pfor gene together with the downregulation of the ldh gene could also explain why a constant level of the lactate concentration is reached before the glucose is totally consumed ( Fig. 8c ). D. vulgaris gene expression studies are not possible in our conditions (using glucose as energy source), as D. vulgaris does not grow in pure culture under these conditions and in consequence no strict control reference can be obtained. Cell interaction between D. vulgaris and C. acetobutylicum appears to be an essential requisite for the increase in H 2 production, as no significant increase was observed when the two bacteria were separated by a membrane ( Fig. 8f ), though in some cases there was a shorter lag, which can be explained by a better anaerobiosis. We show here the establishment in batch culture of a bacterial community constituted of C. acetobutylicum and D. vulgaris , which (i) can grow without a complete set of nutrients essential for growth of D. vulgaris in pure culture, (ii) shows interspecies interaction through physical contact and (iii) allows interspecies exchange of cytoplasmic material. This behaviour permits the emergence of a new phenotype in bacterial communities because it induces modifications of gene expression and changes in metabolism: the mixed community has properties that are not simply the sum of the parts. The physical interaction between the two types of bacteria allows the exchange of molecules of different types and sizes, as different as calcein and GFP or mCherry. Analysis of the genomes of the two bacteria allows us to rule out transport via a type IV secretion system, even modified, as no gene-encoding proteins involved in this secretion type system are detected in the genomes. Moreover, such transport needs specific sequence motifs that are not present in GFP or mCherry [29] , [30] . Transport mechanisms are in general vectorial, but here the interspecies molecular exchange is bidirectional, which could support the idea of connections between cells that allows a free exchange. This type of connection could be more easily established in zones where the peptidoglycan wall is absent or thinner. Cell–cell interaction appears to be an essential requisite for growth of D. vulgaris and the increase in H 2 production, the latter resulting from changes in metabolic fluxes at the pyruvate crossroads, as no growth of D. vulgaris or increase in H 2 production was observed when the two bacteria were separated by a membrane. The absence in the culture medium of substrates necessary for respiratory growth of D. vulgaris appears to be the factor triggering the physical contact between D. vulgaris and C. acetobutylicum as the presence of nutriments, that is, lactate and sulfate, prevents the cell–cell interaction. These results agree with the fact that starvation is an important trigger of stress responses [31] and is often associated with changes in metabolic pathways [32] . It is highly probable that any shortage of nutrients induces a general stress signal in the first stage of growth that here induces interaction. The fact that there is an exchange of molecules between D. vulgaris and E. coli , but not between C. acetobutylicum and E. coli , is compatible with this hypothesis, because E. coli , like C. acetobutylicum , is able to ferment glucose, and is not suffering a nutrient stress condition in the GY medium. The communication between bacteria, which can take several forms [33] , [34] , [35] , [36] , [37] , [38] , is essential for coordinating the behaviour of the whole community. Thus, communication between cells in pure culture regulates the population density by emitting, receiving and responding to a chemical signal, that is, quorum sensing [39] , [40] . Other studies have demonstrated a transfer of outer-membrane proteins between the two strains of Myxococcus xanthus , a wild-type strain acting as donor cell and a mutant strain acting as recipient for the product of the missing gene [41] , [42] . A form of bacterial communication has been described between adjacent cells via connecting ‘nanotubes’, even between Gram-positive and Gram-negative bacteria [23] , which could resemble the cell–cell interaction between C. acetobutylicum and D. vulgaris described here, where we show a bidirectional exchange. In anaerobic systems, it has long been thought that interspecies electron transfer is due to interspecies transfer of H 2 or formate [43] . This is well described in the syntrophic behaviour between SRB and methanogens, where no physical interaction is required because the H 2 produced by the SRB can diffuse freely to be consumed by the methanogens, which act as scavengers [43] , although as any diffusion process, vicinity favours the transfer. Here, on the contrary, tight interaction is indispensable. It is striking that D. vulgaris can grow without lactate and sulfate, but with glucose instead, when in the presence of another type of bacteria that can metabolize glucose, such as C. acetobutylicum (or E. coli ). Which nutrients does D. vulgaris use in the co-culture? Whatever they are, they must come from C. acetobutylicum because only C. acetobutylicum can use glucose. An attractive possibility is that molecules from C. acetobutylicum could act as electron acceptors, replacing sulfate. As we have shown that proteins can be transferred from D. vulgaris to C. acetobutylicum , it may be that electron shuttles such as ferredoxins could act as electron acceptors in D. vulgaris and electron donors in C. acetobutylicum. This could result in the production of additional H 2 . This hypothesis is compatible with the fact that D. vulgaris does not grow when physical interactions are blocked. Several authors have demonstrated that direct electron transfer might also take place through nanowires [44] , [45] , [46] , [47] and it seems to be the primary way of electron transfer in some methanogenic environments. However, proteins known to be involved in this process are absent from D. vulgaris and C. acetobutylicum . The strategy developed by the bacteria in the present case is different and consists in an energetic coupling involving tight physical interactions and transfer of cytoplasmic molecules with C. acetobutylicum (or E. coli ), and this energetic coupling occurs only in the absence of D. vulgaris respiratory substrates. It appears that the type of communication established depends on the environmental conditions and the type of partners involved. Here we demonstrate that another strategy, different from ‘classical’ syntrophy, exists for bacteria and allows them to grow in the absence of substrate. The significant increase in H 2 production in the mixed community arose without any genetic engineering. This is striking, as increases in H 2 yield normally require artificial construction of several mutants that disrupt competing metabolic pathways [48] , [49] . Interestingly, the variation in gene expression developed by our co-culture is the same strategy that a biotechnologist would follow: inactivation of pathways that drain the pyruvate pool. So, despite the uncertainty about the mechanisms behind the changes in gene expression, the establishment of bacterial communities with interaction similar to that between C. acetobutylicu m and D. vulgaris could provide a route for improving biotechnological strategies, as it allows significant modifications of gene expression without genetic engineering. This sort of ecological or community engineering of microbial ecosystems could be the tool that biotechnology needs to develop. Furthermore, the close interaction allowing the exchange of cellular molecules, including proteins, between the bacteria as different as D. vulgaris and C. acetobutylicum , or D. vulgaris and E. coli , which allows the survival of D. vulgaris in the absence of its nutrients and the establishment of a consortium, suggests that bacteria can behave as multicellular organisms in conditions of stress that are closer to what happens in nature, where the availability of nutrients varies considerably. The recent results obtained by Pande et al . [50] revealing nanotubular structures allowing amino acid exchange are along the same line of our observations and support the idea that conditions of nutritional stress can induce cell-cell interactions. Bacterial strains D. vulgaris was from NCIMB 8303 and C. acetobutylicum ATCC824 was kindly supplied by C. Tardif (LCB, UMR7283 CNRS-AMU, Marseilles). Media and growth conditions Strains were grown to steady state in Hungate tubes under anaerobic conditions, in Starkey medium [10] for D. vulgaris and 2YTG medium for C. acetobutylicum [17] . The growth medium (glucose–yeast extract (GY) medium) used for studying the consortium was prepared with glucose (14 mM) and 0.1% yeast extract, and supplemented with the similar inorganic nutrients used for the Starkey preparation (MgCl 2 instead of MgSO 4 ). GY medium was inoculated (10%) with either washed D. vulgaris or C. acetobutylicum , or with the two strains to constitute an artificial consortium in a 1:1 ratio according to the absorbance at 600 nm. In some cases, the medium of growth was supplemented with 20 mM lactate or/and 20 mM sulfate. Some experiments were carried out with a dialysis membrane (molecular mass cutoff of 7 kDa) to physically isolate the two partners. One of the two bacteria, that is, D. vulgaris or C. acetobutylicum , was placed into a dialysis tube and the other outside the dialysis tube. Controls were carried out with one type of bacterium in the dialysis tube and only medium outside. To test the viability of the cells after growth in the GY medium, as single cultures or the co-culture, the specific medium of each bacterium was used and the growth was followed under anaerobic conditions. The sustainability of the co-culture was explored by taking an inoculum after 30 h of culture in GY medium and incubating it again in GY medium. After two transfers, D. vulgaris and C. acetobutylicum still coexisted. The experiments were carried out at least in triplicate. H 2 S concentration was determined as described in Giuliani et al . [51] Real-time qPCR After extraction of genomic DNA from D. vulgaris and C. acetobutylicum using the Wizard Genomic DNA Purification Kit (Promega), DNA purity and concentration were determined and the number of copies was determined by qPCR as described by Savichtcheva et al . [52] The primers used for the qPCR ( dsrA and endoG ) are listed in Supplementary Table 2 . The reaction was performed with a Kit BioRad SsoFast Eva green Super Mix 2 × . The qPCR was carried out in CFX 96 BioRad as follows: 2 min 30 s at 98 °C for initial activation of enzymes, 45 cycles of 5 s at 98 °C, 10 s at 58 °C and 2 s at 72 °C. Experiments were made in triplicate. Reverse transcription PCR Reverse transcription PCR was performed according to Fiévet et al . [53] for estimating the level of expression of genes coding pyruvate ferredoxin oxidoreductase and lactate dehydrogenase. Ten micrograms of total extracted RNA was reverse transcribed with random hexamers. Real-time PCR was carried out on a LightCyclerFastStart DNA MasterPlus SYBR green I Kit (Roche Diagnostics). Complementary DNA was mixed with 0.25 μM of each primer and 2 μl of ‘master mix’ in a final volume of 10 μl. The primer pairs used to quantify different gene expression levels are shown in Supplementary Table 3 . Fluorescence was measured at the end of each amplification step and continuously during the melting curve analysis. Experiments were made in triplicate. Chemical analysis of glucose and metabolites Glucose and lactate were determined by high-performance liquid chromatography (sensitivity 50 mg l −1 ). The compounds were separated using an Aminex HPX-87H, 300 × 7.8 mm column (Bio-Rad). The column temperature was maintained at 35 °C and the flow rate at 0.4 ml min −1 . Organic acids (acetate and butyrate) were determined by gas chromatography (GC-3900, Varian) equipped with a flame ionization detector (sensitivity 20 mg l −1 ) as described by Quéméneur et al . [54] Analysis of biogas production H 2 and CO 2 were quantified in the headspace by gas chromatography (Agilent 4890D) equipped with thermal conductivity detector. The gases were separated using a column GS-CARBONPLOT (30 m × 0.535 mm × 3.00 μm), the injector temperature was 80 °C, the oven temperature was 40 °C and the detector temperature was 90 °C. The carrier gas was N 2 at high purity. Labelling with green or red fluorescent protein The gfp and mCherry ORFs were amplified using the 5′- GAAACCGGTAAAACAAAGGAGGACGTTTATGGTGAGCAAGGGCGAGG -3′ GFP-Fwd, 5′- GATCGATGGTACCTTACTTGTACAGCTCGTCC -3′ GFP-Rev and 5′- GAAACCGGTAAAACAAAGGAGGACGTTTATGGTGAGCAAGGGCGAGGAG -3′ mCherry-pB-Fwd, 5′- GATCGATGGTACCTTACTTGTACAGCTCGTCCATGCC -3′ mCherry-pB-Rev primers, respectively. The PCR amplification of gfp and mCherry was digested and introduced into the AgeI and KpnI sites of pBGF4 plasmid under the control of the hydrogenase constitutive strong promoter as already described [55] to obtain pRD2 and pRD3 plasmids containing gfp and mCherry, respectively. Both are non-stable plasmids in C acetobutylicum . These different plasmids allowed the high expression of gfp and mCherry gene. The DNA sequences were analysed by DNA sequencing (Cogenics, France). Next, pRD2 or pRD3 plasmid was electroporated into the D. vulgaris cells or transformed in E. coli DH10B. Electroporations were carried out as described by Bender et al . [55] with minor modification. D. vulgaris cells were grown in Starkey medium to an optimal absorbance of 0.6 at 600 nm. Cells were harvested by centrifugation and washed with 50 ml of chilled, sterile electroporation wash buffer (30 mM Tris-HCl buffer at pH 7.2, not anaerobic). The resulting pellet was resuspended in 0.5 ml of chilled wash buffer. To 75 μl of cells, 5 μl (4 μg) of plasmid was added and gently mixed. The mixture was transferred to a 2-mm-gap electroporation cuvette (Molecular Bioproducts, San Diego, CA) and introduced to Gene Pulser MXcell system (Bio-Rad, France). The parameters for the electroporation were 1.75 kV, 25 μF and 250 Ω. The electroporated cells were diluted in 1 ml of anaerobic Starkey medium and incubated overnight at 37 °C. One hundred to two hundred microlitres of overnight culture were plated in solid Starkey medium containing gentamycin. The plates were incubated anaerobically for 3–5 days at 37 °C until gentamycin-resistant transformant colonies were visible. Labelling with calcein–AM ester Calcein–AM ester is a small non-fluorescent derivative of calcein that is useful for differentiating between live and dead cells as is sufficiently hydrophobic to pass readily through cell membranes. Once it is inside, esterases cleave the AM groups, yielding the more hydrophilic calcein (623 Da), which is unable to cross membranes and is sequestered in the cytoplasm [56] . The loss of the acetomethoxy group also enables calcein to readily bind intracellular calcium, resulting in a strong yellowish–green fluorescence. D. vulgaris cells were grown in Starkey medium [10] under anaerobic conditions and exponentially growing D. vulgaris (5 ml) was harvested at room temperature by centrifugation at 4,000 g for 10 min, washed twice with Starkey medium and resuspended in 5 ml fresh Starkey medium. Hundred microlitres of calcein–AM ester (1 mg ml −1 in dimethylsulfoxide) were then added to the medium. The suspension was incubated in the dark at 37 °C for 2 h under anaerobic conditions. Cells were subsequently harvested and washed three times in fresh, dye-free GY medium and used in the exchange experiments. The same protocol used for labelling D. vulgaris was followed to label C. acetobutylicum except that C. acetobutylicum cells were grown in 2YTG medium instead of Starkey. Study of exchange of cytoplasmic molecules To study the molecular exchange between the two bacteria, D. vulgaris labelled were mixed with C . acetobutylicum unlabelled or D. vulgaris unlabelled were mixed with C . acetobutylicum labelled in 1:1 ratio according to the absorbance at 600 nm. In some cases, C. acetobutylicum labelled with calcein were mixed with D. vulgaris or E. coli labelled with mCherry. In some other cases, D. vulgaris labelled with calcein were mixed with E. coli labelled with mCherry. The mixture was diluted in 5 ml fresh GY medium and put in a tube containing a coverslip and incubated at 37 °C for 24 h. The coverslip was removed after 24 h of growth and the bacterial cells attached to the coverslip were visualized by fluorescence confocal microscopy. Epifluorescence microscopy Labelling of plasmic membrane and peptidoglycan of C. acetobutylicum and D. vulgaris . To investigate a possible point of contact between D. vulgaris and C. acetobutylicum in the co-culture, the cytoplasmic membrane was marked with FM4-64 fluorochrome ( N -(3- triethylammoniumpropyl)-4-(6-(4-(diethylamino) phenyl) hexatrienyl) pyridinium dibromide) and the peptidoglycan with WGA-FITC fluorochrome (wheat-germ agglutinin). The slides were observed using an automated inverted epifluorescence microscope TE2000-E-PFS (Nikon) and the images were captured with a camera CoolSNAP HQ 2 (Roper Scientific) and analysed with ImageJ52. Confocal microscopy Determination of the transfer of calcein molecules, GFP and mCherry between C. acetobutylicum and D. vulgaris cells was carried out as follows: images of mixtures of labelled and unlabelled cells were acquired on a laser scanning confocal microscope FV 1000 (Olympus, Japan) using an Olympus UPLSAPO 100 × (numerical aperture: 1.40) oil immersion objective. The excitation was provided by a multi-line argon-ion laser. Calcein and GFP were excited at 488 nm and mCherry at 543 nm. The microscope was controlled using Olympus Flu view 2.0c software Scanning electron microscopy SEM was used to visualize in more detail a possible physical contact between D. vulgaris and C. acetobutylicum in the co-culture. The coverslips were immersed in the GY medium before sterilization. During the growth, the coverslips were removed at different times of growth and treated as described by Dubey and Ben-Yehuda [23] , except for the last step of treatment, when they were dried chemically with hexamethyldisilazane for 30 min. Samples were then sputter-coated with gold and palladium (10 nm) with a FINE COAT-ion sputter JFC 1100 and examined using a field-emission gun SEM (JEOL FEGSEM 6320F). Digital images were acquired with the NEWTEC System. How to cite this article: Benomar, S. et al . Nutritional stress induces exchange of cell material and energetic coupling between bacterial species. Nat. Commun. 6:6283 doi: 10.1038/ncomms7283 (2015).